Functional evaluation of autism-associated mutations in NHE9 NHE9 ( SLC9A9 ) is an endosomal cation/proton antiporter with orthologues in yeast and bacteria. Rare, missense substitutions in NHE9 are genetically linked with autism but have not been functionally evaluated. Here we use evolutionary conservation analysis to build a model structure of NHE9 based on the crystal structure of bacterial NhaA and use it to screen autism-associated variants in the human population first by phenotype complementation in yeast, followed by functional analysis in primary cortical astrocytes from mouse. NHE9-GFP localizes to recycling endosomes, where it significantly alkalinizes luminal pH, elevates uptake of transferrin and the neurotransmitter glutamate, and stabilizes surface expression of transferrin receptor and GLAST transporter. In contrast, autism-associated variants L236S, S438P and V176I lack function in astrocytes. Thus, we establish a neurobiological cell model of a candidate gene in autism. Loss-of-function mutations in NHE9 may contribute to autistic phenotype by modulating synaptic membrane protein expression and neurotransmitter clearance. Autism spectrum disorders (ASDs) have emerged as a major public health concern, with an estimated prevalence of 1:88 (ref. 1 ). Characterized by impaired language and social communication, and stereotyped or repetitive behaviours, autism also shows significant comorbidity with intellectual disability (ID) and epilepsy [2] . Although ASD is considered to be the most inheritable of neuropsychiatric disorders, the identification of candidate genes has been complicated by the extreme genetic heterogeneity of the disorder and the prevalence of de novo mutations not found in recent ancestry. Thus, ASD probably involves a combination of alleles with low and high penetrance, with no single variant contributing to more than ~1% of the non-syndromic cases [3] . As the majority of mutations affect one allele, gene dosage may have a critical role in the affected pathways. Despite a growing list of suspects garnered from genome-wide association studies, linkage analysis, cytogenetics and DNA microarrays, most genes remain only candidates in the absence of functional validation. The few existing functional studies have spotlighted a common pathway centring on synaptic transmission in the aetiology of ASD, as well as ID and epilepsy [4] . At the tripartite synapse, it has been proposed that altered expression and activity of proteins at pre- and postsynaptic neuronal membranes disrupts the finely tuned balance of excitatory and inhibitory inputs [5] , with the role of astrocytes being less well studied. Neuronal activity and synaptic transmission require precise control of ionic balance, as well as vesicular trafficking to ensure appropriate surface delivery and turnover of synaptic membrane receptors and transporters [6] . A family of intracellular cation/proton exchangers (NHE6-9) residing on endosomal and recycling compartments regulates luminal pH to control vesicular trafficking [7] , [8] , [9] , [10] , [11] , [12] , [13] , [14] . NHE isoforms have been implicated in a range of neuropsychiatric disorders [15] , [16] , [17] , [18] , [19] , [20] , [21] . Genetic approaches have identified the Na + (K + )/H + exchanger NHE9 ( SLC9A9 ) as a candidate gene of interest in attention-deficit hyperactivity disorder (ADHD), addiction and mental retardation [22] , [23] , [24] , [25] , [26] , [27] , [28] , [29] , [30] . Using homozygosity mapping in consanguineous parents, Morrow et al. [29] identified a large deletion upstream from the 5′-end of NHE9, but not in the coding region itself. Subsequent analysis of ASD patients with epilepsy, from unrelated parents, revealed a nonsense mutation that introduced a premature stop codon at Arg423, in the extracellular loop before the last predicted transmembrane segment of NHE9 (ref. 29 ). Similar nonsense mutations in the last extracellular loop have also been identified in NHE1, where they cause slow-wave epilepsy in mice, and in NHE6, in a patient with Angelman-like syndrome associated with mental retardation and epilepsy [19] , [31] . Several rare, non-conservative coding variants, not found in alleles from asymptomatic individuals were identified in ASD patients [29] . Such coding changes were more common in patients with ASD combined with epilepsy, compared with control subjects (5.95% versus 0.63%) [29] . Although these findings are suggestive of a link to autism in the absence of functional analysis, it is not known whether any of these variants could be causal to the disorder. Two other non-synonymous NHE9 mutations were identified in a rat model of ADHD, although the causal link to the disease was not established [30] . It is possible that the variants associated with autism or ADHD represent benign polymorphisms, as additional changes in other genes were not investigated or ruled out. NHE9 represents an ancient subtype of the cation:proton antiporter 1 (CPA1) family whose best-studied member is the yeast orthologue, Nhx1 (ref. 15 ). Localizing to a prevacuolar compartment, Nhx1 exchanges luminal H + for cations (Na + and K + ) to alkalinize endosomal and vacuolar pH [32] . Hyperacidification of compartments from gene deletion or loss-of-function mutations in Nhx1 disrupts cargo delivery to the vacuole and confers growth sensitivity to high salt, acidic pH and the drug hygromycin B, which are all readily quantifiable phenotypes [32] , [33] . Therefore, we used a yeast model for rapid assessment of NHE9 variants as a first approximation of function. The abnormal accumulation of glutamate in the brain of patients with NHE6 mutations is indicative of an underlying problem in glutamate clearance from the synapse [19] . Glutamate is excitotoxic at high concentrations, and aberrant glutamate levels are associated with neurological abnormalities of epilepsy and cerebellar degeneration, both characteristic symptoms of Angelman-like syndrome associated with NHE6 mutations [19] . The bulk of glutamate released into the neuronal synapse is cleared by rapid uptake into astrocytes, the single largest population of cells in the brain [34] . Given the shared clinical symptoms of epilepsy, ID and ASD in patients, it seemed probable that similar to NHE6, NHE9 could regulate glutamate clearance in the synapse. In this study, we provide the first functional analysis of NHE9 in a neurobiological model. We show that altered gene dosage can significantly change vesicular pH and modulate cell surface expression and activity of glutamate transporters in murine cortical astrocytes, where they have the potential to impact neurotransmission. Finally, we extend the functional analysis of autism-associated coding variants in NHE9 from yeast to primary astrocytes to gain novel insight into the aetiology of ASD. All three autism-associated genetic variants in the NHE9 tested were scored as loss-of-function mutations in astrocytes and, therefore, could be causal to disease phenotype. Our study provides crucial functional insight that was lacking from previous genetic analysis and establishes a role for NHE9 in a neurobiological model. A model structure of NHE9 As a first step in determining whether rare coding variants in NHE9 contributed to the autism phenotype, we constructed a structural model of the membrane domain of NHE9, and its yeast orthologue Nhx1, based on the crystal structure of a distantly related bacterial orthologue, NhaA [35] . Previously, we used evolutionary analysis and a composite fold-recognition approach to propose a three-dimensional model structure of NHE1, a prototype of the cation/proton superfamily [36] , [37] . Utilizing a similar methodology, we aligned yeast Nhx1 and mammalian NHE9 to NhaA ( Fig. 1a ), as well as to NHE1. In accordance with phylogenetic clustering, the resulting alignments showed that both Nhx1 and NHE9 were significantly more closely related to NHE1 than to bacterial NhaA, with sequence identities of 30% and 32% for the alignments of Nhx1 and NHE9 to NHE1, respectively, whereas aligning Nhx1 and NHE9 to NhaA resulted in sequence identities of 15% and 14%, respectively. This allowed us to extend the structural model from NHE1 to NHE9 ( Figs 1b and 2a ) and Nhx1 ( Fig. 1c ). To evaluate the Nhx1 and NHE9 models, we examined characteristic traits of membrane proteins, namely the distribution of hydrophobicity and evolutionary conservation. Consistent with the reliability of the models, we show a preponderance of hydrophobic residues within the predicted membrane spans ( Fig. 1b ), and concentration of evolutionarily conserved residues within the core regions of the transporter ( Fig. 2a ). 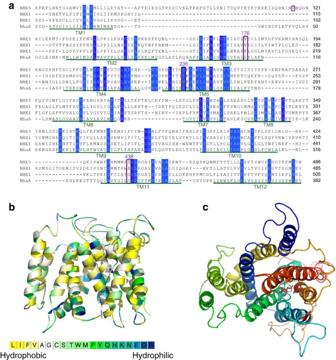Figure 1: Structural modelling of NHE9 and Nhx1. (a) Alignment of the sequences of human NHE9,S. cerevisiaeNhx1, human NHE1 andE. coliNhaA. Transmembrane segments are underlined and numbered. The positions of four NHE9 variants are boxed. (b) Hydrophobicity analysis, using the blue-to-yellow colour code shown in the colour bar of the NHE9 model structure shows that the lipid facing amino acids are (overall) hydrophobic, as they should63. (c) Model structure of yeast Nhx1 showing shared protein fold common to the NHE family, and residues targeted for mutation in red (stick representation). Figure 1: Structural modelling of NHE9 and Nhx1. ( a ) Alignment of the sequences of human NHE9, S. cerevisiae Nhx1, human NHE1 and E. coli NhaA. Transmembrane segments are underlined and numbered. The positions of four NHE9 variants are boxed. ( b ) Hydrophobicity analysis, using the blue-to-yellow colour code shown in the colour bar of the NHE9 model structure shows that the lipid facing amino acids are (overall) hydrophobic, as they should [63] . ( c ) Model structure of yeast Nhx1 showing shared protein fold common to the NHE family, and residues targeted for mutation in red (stick representation). 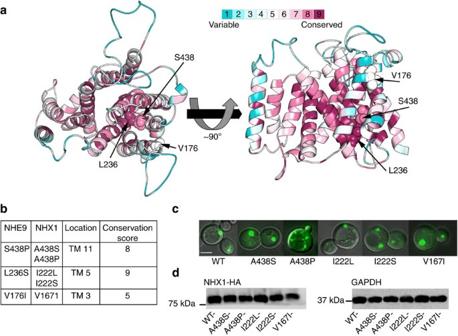Figure 2: Modelling of autism-associated NHE9 variants. (a) Top and side views of a model structure of the membrane domain of NHE9 based on the structure ofE. coliNhaA and coloured according to the degree of ConSurf conservation, with turquoise through maroon, indicating variable through conserved amino acid positions. Three autism-associated variants (S438P, L236S and V176I) are shown in space-filled form. (b) Site-directed mutagenesis was used to introduce equivalent NHE9 mutations into yeast Nhx1 (A438P, I222S and V167I) as well as ‘humanized’ variants A438S and I222L to mimic wild-type NHE9. (c) Nhx1 constructs tagged with GFP were expressed in thenhx1Δ null strain and visualized ( × 100 objective) as fluorescent punctae, characteristic of prevacuolar compartments. Scale bar, 20 μm. (d) Immunoblot analysis with anti-haemagglutinin (anti-HA) was used to detect similar expression levels of HA-tagged Nhx1 and variants. GAPDH (glyceraldehyde-3-phosphate dehydrogenase) was used as loading control. Full size image Figure 2: Modelling of autism-associated NHE9 variants. ( a ) Top and side views of a model structure of the membrane domain of NHE9 based on the structure of E. coli NhaA and coloured according to the degree of ConSurf conservation, with turquoise through maroon, indicating variable through conserved amino acid positions. Three autism-associated variants (S438P, L236S and V176I) are shown in space-filled form. ( b ) Site-directed mutagenesis was used to introduce equivalent NHE9 mutations into yeast Nhx1 (A438P, I222S and V167I) as well as ‘humanized’ variants A438S and I222L to mimic wild-type NHE9. ( c ) Nhx1 constructs tagged with GFP were expressed in the nhx1 Δ null strain and visualized ( × 100 objective) as fluorescent punctae, characteristic of prevacuolar compartments. Scale bar, 20 μm. ( d ) Immunoblot analysis with anti-haemagglutinin (anti-HA) was used to detect similar expression levels of HA-tagged Nhx1 and variants. GAPDH (glyceraldehyde-3-phosphate dehydrogenase) was used as loading control. Full size image Three autism-associated substitutions, namely V176I, L236S and S438P ( Figs 1a and 2a ), reside within the membrane domain of NHE9, in positions that are evolutionarily conserved among all eukaryotic transporters. A fourth mutation, P117T, is localized to a highly variable extracellular loop and could not be modelled with certainty in the yeast orthologue ( Fig. 1a ). Other substitutions resided outside the homology region, including the carboxy-terminal hydrophilic tail. As seen in Fig. 2a , L236 and S438 are highly conserved in all eukaryotic and prokaryotic homologues and buried in the protein core, whereas V176 is only moderately conserved and faces the lipid bilayer. Furthermore, the autism-associated variants L236S and S438P change the physicochemical nature and stereochemistry of the amino acid side chains significantly, whereas the V176I change is moderate. Phenotype screening of autism-associated mutations in yeast Phenotype complementation in yeast offers a rapid and first approach towards functional screening of mutations. The nhx1 Δ-null strain exhibits clearly defined and quantifiable growth defects relating to pH, salt and drug sensitivity that have been linked to ion transport and vesicle trafficking [32] , [33] . Therefore, we introduced autism-associated mutations into equivalent positions in Nhx1 ( Fig. 2b ; A438P, I222S and V167I). As two of these positions carried moderate substitutions in Nhx1, we also generated ‘humanized’ versions, A438S and I222L, equivalent to NHE9. All five substitutions and wild-type Nhx1 were separately tagged with green fluorescent protein (GFP) or haemagglutinin and expressed in nhx1 Δ yeast. Similar to wild-type Nhx1, most mutants were localized to one to two punctate compartments ( Fig. 2c ) previously identified as prevacuolar endosomes [38] , and were expressed at equivalent levels ( Fig. 2d ). Mutant A438P showed a shift in distribution to multiple puncta, suggesting a possible delay in trafficking of the mutant protein to the prevacuolar compartment. Sensitivity to hygromycin B toxicity is increased in nhx1 Δ as a result of defective trafficking to the vacuole, believed to be the site of drug detoxification [32] , [33] . Plasmid expressing wild-type Nhx1 conferred tolerance to hygromycin B growth toxicity ( Fig. 3a ). Similarly, the humanized versions of Nhx1, A438S and I222L were equally effective in protecting against drug toxicity. In contrast, two autism-associated variants, A438P and I222S, closely resembled the vector-transformed null mutant, consistent with complete loss of function. The third variant, V167I, resembled wild-type Nhx1. We obtained similar results with growth sensitivity to high salt ( Fig. 3b ) and to low pH ( Fig. 3c ). In each case the control substitutions, equivalent to those in NHE9, resembled wild type, whereas autism-associated variants A438P and I222S were similar to the vector-transformed nhx1 Δ-null strain. Consistently, the V167I variant showed no loss of function in these growth phenotypes. 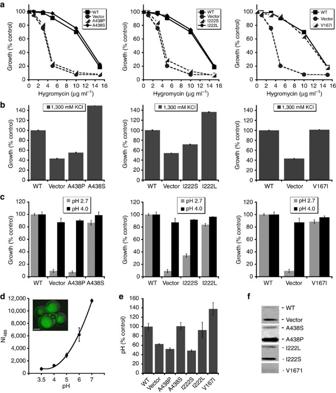Figure 3: Phenotype screening of autism-associated variants in yeast. (a) Growth sensitivity to hygromycin B. Yeastnhx1Δ strains expressing the vector or indicated Nhx1 constructs were inoculated with equal numbers of cells in APG medium (pH 4.0) supplemented with hygromycin B. Growth (OD600) was measured after 17 h at 30 °C and is expressed as the percentage of growth in the absence of hygromycin. (b) Growth sensitivity to KCl. Cultures, as ina, were grown in a medium supplemented with KCl. (c) Growth sensitivity to acidic pH. Cultures, as ina, were grown in APG medium buffered to pH 4.0 or 2.7 for 21 h. Results shown fora–care averages of triplicate determinations and are representative of at least three independent experiments. (d) Measurement of vacuolar pH with BCECF (2′,7′-bis-(2-carboxyethyl)-5(6)-carboxyfluorescein)-acetoxymethyl ester). Cells were loaded with BCECF resulting in accumulation of the dye in yeast vacuoles, as seen in the fluorescent micrograph ( × 100 objective). (d) Inset: scale bar, 20 μm. Fluorescence was normalized to cell number (NI485) and calibrated against vacuolar pH (e). Normalized, pH-sensitive fluorescence as indfor the yeast strains shown. Mean was plotted from at least three independent experiments fordande. All error bars represent s.d. (f) Sorting of CPY. Extracellular CPY in culture supernatants (600 μl) was assessed by slot blots. Samples were applied onto fixed slots by vacuum suction and the nitrocellulose filter treated as in a western blot. Figure 3: Phenotype screening of autism-associated variants in yeast. ( a ) Growth sensitivity to hygromycin B. Yeast nhx1 Δ strains expressing the vector or indicated Nhx1 constructs were inoculated with equal numbers of cells in APG medium (pH 4.0) supplemented with hygromycin B. Growth (OD 600 ) was measured after 17 h at 30 °C and is expressed as the percentage of growth in the absence of hygromycin. ( b ) Growth sensitivity to KCl. Cultures, as in a , were grown in a medium supplemented with KCl. ( c ) Growth sensitivity to acidic pH. Cultures, as in a , were grown in APG medium buffered to pH 4.0 or 2.7 for 21 h. Results shown for a – c are averages of triplicate determinations and are representative of at least three independent experiments. ( d ) Measurement of vacuolar pH with BCECF (2′,7′-bis-(2-carboxyethyl)-5(6)-carboxyfluorescein)-acetoxymethyl ester). Cells were loaded with BCECF resulting in accumulation of the dye in yeast vacuoles, as seen in the fluorescent micrograph ( × 100 objective). ( d ) Inset: scale bar, 20 μm. Fluorescence was normalized to cell number (NI 485 ) and calibrated against vacuolar pH ( e ). Normalized, pH-sensitive fluorescence as in d for the yeast strains shown. Mean was plotted from at least three independent experiments for d and e . All error bars represent s.d. ( f ) Sorting of CPY. Extracellular CPY in culture supernatants (600 μl) was assessed by slot blots. Samples were applied onto fixed slots by vacuum suction and the nitrocellulose filter treated as in a western blot. Full size image Sensitivity to low pH in nhx1 Δ correlates with vacuolar hyperacidification, pointing to Na + (K + )/H + antiport as a major leak pathway for exit of protons transported into the endosome/vacuole by the V-ATPase [32] . We evaluated vacuolar pH in situ by using the pH-sensitive fluorescent dye BCECF-AM, which is de-esterified and sequestered in the vacuolar lumen ( Fig. 3d , inset) [38] allowing fluorescence intensity to be normalized to cell number (NI 485 ) and calibrated to pH ( Fig. 3d ). Vacuolar pH in vector-transformed nhx1 Δ was more acidic relative to wild type, and similar to strains expressing the loss-of-function A438P and I222S variants. In contrast, vacuolar pH in cells expressing variants A438S, 1222L and V167I was more alkaline and similar to wild-type Nhx1 ( Fig. 3e ). A consequence of hyperacidic luminal pH is that Vps10, a chaperone for lysosomal hydrolases, is retained and degraded in the prevacuolar compartment in nhx1 Δ mutants. As a result, cargo destined for the vacuole, including carboxypeptidase Y (CPY), is missorted to the extracellular medium of nhx1 Δ strains [38] , where it can be detected by western analysis of slot blots ( Fig. 3f ). Missorting of CPY to the medium was effectively rescued by plasmids expressing wild-type Nhx1 or humanized variants A48S and I222L. In contrast, extracellular CPY was elevated in autism-associated variants A438P and I222S, similar to the vector-transformed nhx1 Δ host strain. Again, variant V167I phenocopied wild-type Nhx1 in rescuing missorting of CPY to the medium. Taken together, this analysis revealed that substitutions in the evolutionarily conserved sites on Nhx1, orthologous to autism-associated variants S438P and L236S in NHE9, lead to loss of function, whereas a substitution in a variable region predicted to face the lipid bilayer, equivalent to V176I in NHE9, retained function in yeast Nhx1. Expression and developmental regulation of NHE9 in brain In the wake of the association of NHE9 with autism, we sought to investigate the spatiotemporal distribution of NHE9 in the developing and adult mouse brain. Although no single region of the brain has yet been clearly identified as being associated with autism, two decades of magnetic resonance imaging studies have implicated the cerebellum, frontal cortex, hippocampus and amygdala. Post-mortem findings, animal models and neuroimaging studies further strengthen these observations [39] , [40] . In-situ hybridization data of the adult mouse brain obtained from the Allen Brain Atlas [41] indicate that the expression levels of NHE9 are highest in the cortex (~27% of total NHE9 expression in the brain), hippocampus (~30%) and the olfactory lobes (~50%; Fig. 4a ) compared with the other regions of the brain. Variations of gene expression in the brain may have a crucial role in the behavioural phenotypes observed in autism and suggest a strong association with the cortex, which is the seat of memory, attention, thought, language and consciousness in the brain. Recent reports comparing autistic and control brains suggested an attenuation of normal differential gene expression between frontal and temporal cortex in autistic brains [42] . Moreover, as autism is a neurodevelopmental disorder we expect NHE9 to have a functional role during development. Indeed, in-situ hybridization data of the developing mouse brain [43] revealed differential expression of NHE9 during the various stages of development ( Fig. 4b ). NHE9 expression was consistently high in the prosomere 1 (p1) region of the diencephalon in the embryonic forebrain ( Fig. 4c ). In addition to the forebrain, expression levels of NHE9 were also high in the midbrain by postnatal day 4. Although the p1 and midbrain showed high levels of NHE9 expression in postnatal day-28 pups, highest levels of NHE9 were observed in the telencephalic vesicle of the forebrain. The pontomedullary region of the hindbrain also showed NHE9 expression comparable to the p1 region by postnatal day 28. Finally, the adult brain is primarily composed of two broad classes of cells: neurons and glial cells. We compared the mRNA transcript levels of NHE9 in neurons and astrocytes, the most abundant macroglial cells in the cortex. NHE9 expression was ~1.2-fold higher in astrocytes relative to the neurons ( Fig. 4d ). 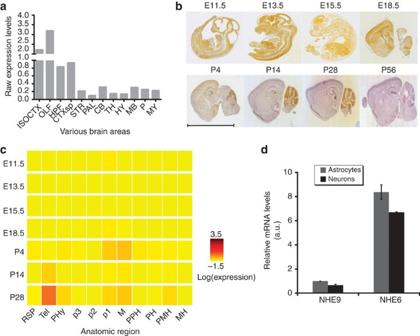Figure 4: Developmental regulation of NHE9 in mouse and expression in primary brain cells. (a) Raw expression levels of NHE9 in various regions of the mouse brain determined fromin-situhybridization (ISH) data obtained from Allen Brain Atlas (available from:http://mouse.brain-map.org/). ISOCTX, isocortex; OLF, olfactory areas; HPF, hippocampal formation; CTXsp, cortical subplate; STR, striatum; PAL, pallidum; CB, cerebellum; TH, thalamus; HY, hypothalamus; MB, midbrain; P, pons; MY, medulla. (b) NHE9 gene expression in developing mouse brain characterized by ISH in sagittal plane across four embryonic and three early postnatal ages. Feulgen-HP yellow DNA counterstain, a nuclear stain, was used to add definition to the tissue. This counterstain is used in conjunction with ISH for all data shown except for P56, to provide tissue context to the ISH signal, which is otherwise difficult to discern due to the very light tissue background for embryonic ISH. Images were obtained from the Allen Institute for Brain Science, Allen Developing Mouse Brain Atlas (available from:http://developingmouse.brain-map.org) (c) ISH data showing expression summary of NHE9 in the various regions of the mouse brain during development, obtained from the Allen Developing Mouse Brain Atlas (available from:http://developingmouse.brain-map.org). RSP, rostral secondary prosencephalon; Tel, telencephalic vesicle; PHy, peduncular (caudal) hypothalamus; p3, prosomere 3; p2, prosomere 2; p1, prosomere 1; M, midbrain; PPH, prepontine hindbrain; PH, pontine hindbrain; PMH, pontomedullary hindbrain; MH, medullary hindbrain. Scale bar, 3168 μm. (d) Quantitative PCR analysis of NHE6 and NHE9 in primary murine neurons and astrocytes with mRNA normalized to two reference genes (GAPDHand 18S RNA) and expressed relative to NHE9 mRNA level. Error bars represent s.d. determined from triplicate measurements. Figure 4: Developmental regulation of NHE9 in mouse and expression in primary brain cells. ( a ) Raw expression levels of NHE9 in various regions of the mouse brain determined from in-situ hybridization (ISH) data obtained from Allen Brain Atlas (available from: http://mouse.brain-map.org/ ). ISOCTX, isocortex; OLF, olfactory areas; HPF, hippocampal formation; CTXsp, cortical subplate; STR, striatum; PAL, pallidum; CB, cerebellum; TH, thalamus; HY, hypothalamus; MB, midbrain; P, pons; MY, medulla. ( b ) NHE9 gene expression in developing mouse brain characterized by ISH in sagittal plane across four embryonic and three early postnatal ages. Feulgen-HP yellow DNA counterstain, a nuclear stain, was used to add definition to the tissue. This counterstain is used in conjunction with ISH for all data shown except for P56, to provide tissue context to the ISH signal, which is otherwise difficult to discern due to the very light tissue background for embryonic ISH. Images were obtained from the Allen Institute for Brain Science, Allen Developing Mouse Brain Atlas (available from: http://developingmouse.brain-map.org ) ( c ) ISH data showing expression summary of NHE9 in the various regions of the mouse brain during development, obtained from the Allen Developing Mouse Brain Atlas (available from: http://developingmouse.brain-map.org ). RSP, rostral secondary prosencephalon; Tel, telencephalic vesicle; PHy, peduncular (caudal) hypothalamus; p3, prosomere 3; p2, prosomere 2; p1, prosomere 1; M, midbrain; PPH, prepontine hindbrain; PH, pontine hindbrain; PMH, pontomedullary hindbrain; MH, medullary hindbrain. Scale bar, 3168 μm. ( d ) Quantitative PCR analysis of NHE6 and NHE9 in primary murine neurons and astrocytes with mRNA normalized to two reference genes ( GAPDH and 18S RNA) and expressed relative to NHE9 mRNA level. Error bars represent s.d. determined from triplicate measurements. Full size image Functional expression and localization of NHE9 in astrocytes Astrocytes are critical for the long-term modulation of neuronal synapses, as well as acute clearance of the excitatory neurotransmitter, glutamate, from the synaptic cleft [34] . In animal models of autism, astrocytic clearance of glutamate is altered and glutamate transporter levels decreased [44] . Elevated levels of glutamate in the synapse trigger seizures, and seizures are well known to be comorbid with autism. As shown by Morrow et al. [29] , a significant subset of NHE9 variants was associated with both autism and seizures. Furthermore, elevated brain glutamate levels are observed in patients with mutations in the closely related orthologue NHE6 (ref. 19 ). Therefore, to confirm our findings in yeast and extend the analysis of autism-associated variants in NHE9 to a neurobiological model, we evaluated function in astrocytes [19] . We began by evaluating expression levels of NHE9 and NHE6 isoforms in primary mouse astrocytes. Transcript analysis revealed the presence of both NHE6 and NHE9 in complementary DNA extracts from astrocytes ( Fig. 5a ), as well as in neurons ( Fig. 4d ). Knockdown of NHE9 (by ~80%) in the astrocytes did not alter transcript levels for NHE6, although a modest compensatory increase in NHE9 levels (15%, P =0.004; Student’s t -test, n =three biological replicates) was consistently observed upon knockdown of NHE6 ( Fig. 5b ). We also engineered lentiviral-mediated overexpression of NHE9-GFP ( Fig. 5b ). NHE9-GFP colocalized in part with markers for the early endosome EEA1 (fractional colocalization, 0.11±0.06 s.d., n =46) and more extensively with the recycling endosome marker Rab11 (0.46±0.25 s.d., n =71) by immunofluorescence ( Fig. 5c,d , top and middle panel). No NHE9-GFP was observed in the late endosome, as evidenced by lack of colocalization with lysobisphosphatidic acid (−0.01±0.02 s.d., n =50; Fig. 5c,d , bottom panel). 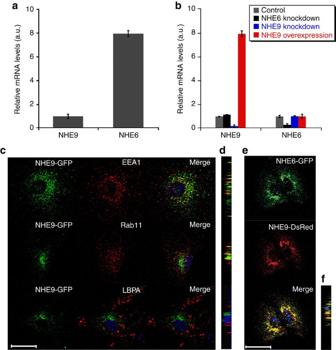Figure 5: Subcellular localization and functional analysis of NHE9. (a) Quantitative PCR (qPCR) analysis of NHE6 and NHE9 mRNA in primary cortical astrocytes, normalized to two reference genes (GAPDHand 18S RNA) and expressed relative to NHE9 mRNA level. Error bars represent s.d. determined from triplicate measurements. Baseline expression of NHE9 is significantly lower than NHE6 (note that the eightfold difference corresponds to three cycles of PCR amplification on Log2scale). (b) qPCR analysis showing the efficacy of overexpression of (NHE9) and short hairpin RNA knockdown (NHE9 and NHE6) in primary astrocyte culture. The data are plotted as average fold change of mRNA levels relative to control levels, with s.d. determined from triplicate measurements. (c) Subcellular localization of NHE9 in primary cultured cortical astrocytes determined by immunofluorescence confocal microscopy ( × 63 objective) after fixation with 4% paraformaldehyde. Top, NHE9-GFP (green) partly localizes with early endosome marker, EEA1 (red) as seen in the Merge. Middle, NHE9-GFP (green) partly localizes with recycling endosome marker, Rab11 (red) as seen in the Merge. Bottom, NHE9-GFP (green) does not localize with late endosome marker, LBPA (red). (d) Orthogonal views of subcellular localization of NHE9 from merged images inc. (e) Overlapping subcellular localization of NHE6-GFP (green) and NHE9-DsRed (red) in primary cultured cortical astrocytes, as seen in Merge and (f) orthogonal view. Scale bars, 50 μm (forcande). Figure 5: Subcellular localization and functional analysis of NHE9. ( a ) Quantitative PCR (qPCR) analysis of NHE6 and NHE9 mRNA in primary cortical astrocytes, normalized to two reference genes ( GAPDH and 18S RNA) and expressed relative to NHE9 mRNA level. Error bars represent s.d. determined from triplicate measurements. Baseline expression of NHE9 is significantly lower than NHE6 (note that the eightfold difference corresponds to three cycles of PCR amplification on Log 2 scale). ( b ) qPCR analysis showing the efficacy of overexpression of (NHE9) and short hairpin RNA knockdown (NHE9 and NHE6) in primary astrocyte culture. The data are plotted as average fold change of mRNA levels relative to control levels, with s.d. determined from triplicate measurements. ( c ) Subcellular localization of NHE9 in primary cultured cortical astrocytes determined by immunofluorescence confocal microscopy ( × 63 objective) after fixation with 4% paraformaldehyde. Top, NHE9-GFP (green) partly localizes with early endosome marker, EEA1 (red) as seen in the Merge. Middle, NHE9-GFP (green) partly localizes with recycling endosome marker, Rab11 (red) as seen in the Merge. Bottom, NHE9-GFP (green) does not localize with late endosome marker, LBPA (red). ( d ) Orthogonal views of subcellular localization of NHE9 from merged images in c . ( e ) Overlapping subcellular localization of NHE6-GFP (green) and NHE9-DsRed (red) in primary cultured cortical astrocytes, as seen in Merge and ( f ) orthogonal view. Scale bars, 50 μm (for c and e ). Full size image To investigate the effect of altered NHE9 levels on luminal pH in recycling endosomes, we took advantage of the excellent overlap in localization with transferrin (Fig. 7b, top panel), following 60-min uptake into live cells. Fluorescence ratio imaging was done by using a combination of pH-sensitive fluorescein isothiocyanate-tagged transferrin with pH-insensitive Alexa Fluor-tagged transferrin as control for transferrin loading, and the endosomal pH was determined from a calibration curve ( Fig. 6a ). Relative to the control cells (pH 5.7±0.22), endosomal pH in NHE9-overexpressing cells was more alkaline (pH 6.39±0.054), as expected from Na + (K + )/H + exchange mediating proton leak from the endosomes ( Fig. 6b ). These results are consistent with increased endosomal pH observed by Nakamura et al. [8] in COS7 cells overexpressing NHE9. Although luminal pH decreased upon knockdown of NHE9 (to pH 5.39, P =0.08; Student’s t -test, n =three biological replicates; Fig. 6b ), the difference fell short of significance. Therefore, we examined the effect of NHE9 knockdown in primary cultured human glioma cells ( Fig. 6c ). We did observe significant acidification of endosomes upon NHE9 knockdown (pH 6.60, P <0.05; Student’s t -test, n =three biological replicates) relative to control (pH 6.88). These results suggest functional differences between mouse and human astrocyte cells, consistent with the limitations of the mouse model in recapitulating human disease. It is possible that NHE6 compensates for loss of NHE9 in mouse cortical astrocytes. Indeed, we observed high levels of colocalization of NHE6-GFP and NHE9-DsRed in murine astrocytes ( Fig. 5e,f ), consistent with redundant roles for NHE6 and NHE9 in regulating endosomal pH. 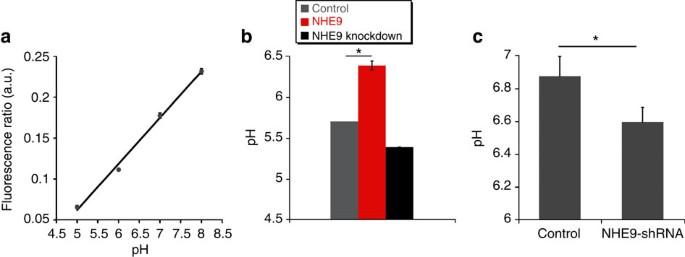Figure 6: NHE9 regulates endosomal pH. (a) Calibration of endosomal pH from fluorescence ratio of internalized transferrin (Tf)–fluorescein isothiocyanate (FITC) and Tf-Alexafluor. Cells were loaded with tagged Tf for 1 h, then exposed to nigericin (100 μM) and pH defined medium (pH 5.0 to pH 8.0). Internalized Tf was quantified using flow cytometry. (b) NHE9 expression alkalinizes endosomal lumen. pH of Tfn-positive endosomes in primary cultured cortical astrocytes was determined in control, NHE9 overexpression and NHE9 short hairpin RNA (shRNA) knockdown conditions. Results are averages of three biological replicates, each done in triplicate (*P<0.05). (c) Knockdown of NHE9 acidifies Tfn-positive endosomes in primary cultured human glioma cells. Results are averages of three replicates (*P<0.05). Statistical analysis was by Student’st-test; all error bars represent s.d. Figure 6: NHE9 regulates endosomal pH. ( a ) Calibration of endosomal pH from fluorescence ratio of internalized transferrin (Tf)–fluorescein isothiocyanate (FITC) and Tf-Alexafluor. Cells were loaded with tagged Tf for 1 h, then exposed to nigericin (100 μM) and pH defined medium (pH 5.0 to pH 8.0). Internalized Tf was quantified using flow cytometry. ( b ) NHE9 expression alkalinizes endosomal lumen. pH of Tfn-positive endosomes in primary cultured cortical astrocytes was determined in control, NHE9 overexpression and NHE9 short hairpin RNA (shRNA) knockdown conditions. Results are averages of three biological replicates, each done in triplicate (* P <0.05). ( c ) Knockdown of NHE9 acidifies Tfn-positive endosomes in primary cultured human glioma cells. Results are averages of three replicates (* P <0.05). Statistical analysis was by Student’s t -test; all error bars represent s.d. Full size image Evaluation of autism-associated NHE9 mutations in astrocytes Synaptic function is modulated by targeting and recycling of transporters and receptors to and from the astrocyte cell surface [45] . In the yeast model, Nhx1-mediated regulation of endosomal pH is critical for cell surface expression and turnover of membrane proteins. Therefore, we investigated whether NHE9 knockdown or overexpression similarly altered the function and expression of cell surface receptors and transporters in astrocytes. Steady-state levels of fluorescence-tagged transferrin were significantly elevated (by 1.75-fold) in astrocytes overexpressing NHE9 (Fig. 8a,c), with corresponding stabilization of the transferrin receptor, observed upon blocking protein synthesis by cycloheximide addition (Fig. 8b). Although internalized transferrin levels were not decreased upon knockdown of endogenous NHE9, treatment with short hairpin RNA effectively reversed the elevation seen in NHE9-overexpressing cells (Fig. 8c). We used this gain-of-function phenotype to assess the three autism-associated variants in NHE9. GFP-tagged variants, L236S, S438P and V176I, were expressed at levels equivalent to wild-type NHE9 in primary astrocytes ( Fig. 7a ) and individually colocalized with Alexa Fluor-labelled transferrin ( Fig. 7b ). After incubation with Alexa-633-transferrin for 1 h at 37 °C, none of the three variants displayed elevated levels of intracellular transferrin, resembling the vector-transformed control ( Fig. 8d ). Unexpectedly, this included the V176I variant that retained function in the yeast model. 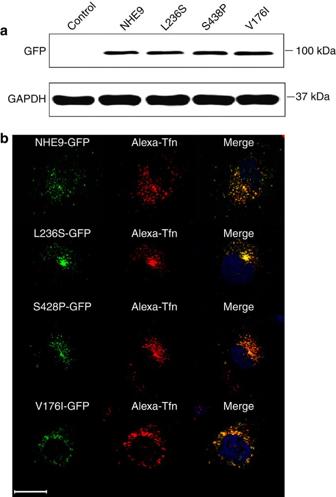Figure 7: Expression and localization of NHE9 variants in primary astrocytes. (a) Expression levels of NHE9 and autism-associated polymorphisms are similar in primary astrocytes. Immunoblot of total primary astrocyte cell lysate (100 μg) from Control (empty vector transfection) and cells expressing NHE9-GFP, L236S-GFP, S438P-GFP and V176IGFP using anti-GFP antibody. (b) Localization of NHE9 and autism-associated variants to transferrin-positive endosomes in primary astrocytes. Confocal fluorescence images ( × 63 objective) of GFP-tagged NHE9 and indicated patient polymorphisms (green) localize with Alexa Fluor-tagged transferrin after 55 min of uptake (red), as described in the Methods. Significant colocalization can be seen in merged images by the presence of yellow puncta. Scale bar, 50 μm. Figure 7: Expression and localization of NHE9 variants in primary astrocytes. ( a ) Expression levels of NHE9 and autism-associated polymorphisms are similar in primary astrocytes. Immunoblot of total primary astrocyte cell lysate (100 μg) from Control (empty vector transfection) and cells expressing NHE9-GFP, L236S-GFP, S438P-GFP and V176IGFP using anti-GFP antibody. ( b ) Localization of NHE9 and autism-associated variants to transferrin-positive endosomes in primary astrocytes. Confocal fluorescence images ( × 63 objective) of GFP-tagged NHE9 and indicated patient polymorphisms (green) localize with Alexa Fluor-tagged transferrin after 55 min of uptake (red), as described in the Methods. Significant colocalization can be seen in merged images by the presence of yellow puncta. Scale bar, 50 μm. 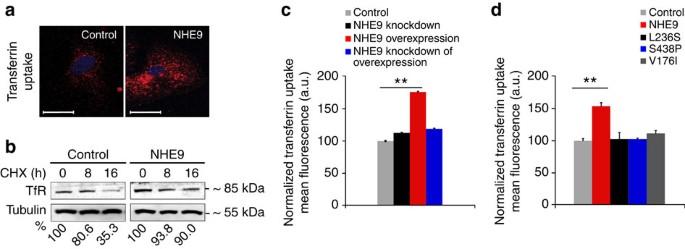Figure 8: Functional differences between NHE9 and variants revealed by transferrin uptake. (a) Maximum projection confocal images ( × 63 objective) showing steady-state Tfn-Alexa Fluor uptake in control (left) and NHE9-GFP-expressing astrocytes (right). Scale bars, 50 μm (b) Immunobottings, using anti-TfR antibody, showing the effects of 100 μM cycloheximide (CHX) on TfR in control and NHE9-GFP-expressing cells. TfR bands were normalized to Tubulin levels and expressed as percentage of controls lacking CHX. (c) Steady-state Tfn-Alexa Fluor uptake was significantly elevated (**P<0.005; Student’st-test,n=three biological replicates) upon NHE9-GFP expression and reversed upon subsequent knockdown in the same cells. (d) Steady-state uptake of Tfn-Alexa Fluor in astrocytes expressing wild-type NHE9-GFP or three autism-association variants. Variants (L236S, S438P and V176I) failed to elevate Tfn-Alexa Fluor uptake, showing a loss-of-function phenotype (n=three biological replicates). Error bars (c,d) represent s.d. **P<0.005. Full size image Figure 8: Functional differences between NHE9 and variants revealed by transferrin uptake. ( a ) Maximum projection confocal images ( × 63 objective) showing steady-state Tfn-Alexa Fluor uptake in control (left) and NHE9-GFP-expressing astrocytes (right). Scale bars, 50 μm ( b ) Immunobottings, using anti-TfR antibody, showing the effects of 100 μM cycloheximide (CHX) on TfR in control and NHE9-GFP-expressing cells. TfR bands were normalized to Tubulin levels and expressed as percentage of controls lacking CHX. ( c ) Steady-state Tfn-Alexa Fluor uptake was significantly elevated (** P <0.005; Student’s t -test, n =three biological replicates) upon NHE9-GFP expression and reversed upon subsequent knockdown in the same cells. ( d ) Steady-state uptake of Tfn-Alexa Fluor in astrocytes expressing wild-type NHE9-GFP or three autism-association variants. Variants (L236S, S438P and V176I) failed to elevate Tfn-Alexa Fluor uptake, showing a loss-of-function phenotype ( n =three biological replicates). Error bars ( c , d ) represent s.d. ** P <0.005. Full size image A function specific to astrocytes at the excitatory synapse is clearance of excess glutamate. We therefore investigated the effect of NHE9 and its variants on glutamate uptake in astrocytes. GLAST (GLutamate ASpartate Transporter) is a high-affinity, Na + -dependent glutamate transporter highly expressed in astrocytes [46] , where it partially colocalizes with endosomal NHE9 ( Fig. 9a–d ). Overexpression of NHE9 resulted in ~1.9-fold increase in 3 H-glutamate uptake relative to control cells, whereas all three autism-associated variants were similar to vector-transformed control ( Fig. 9e ). Although total amounts remained unchanged in all cell lines, surface expression of GLAST transporter increased by approximately twofold in astrocytes expressing wild-type NHE9 but not the autism-associated variants L236S, S438P and V176I ( Fig. 9f,g ). Consistent with these observations, alkalinization of the transferrin-positive endosomal compartment was only observed in cells expressing wild-type NHE9 ( Fig. 10a,b ). Taken together, our findings indicate that all three autism-associated variants were associated with loss-of-function phenotypes in astrocytes. 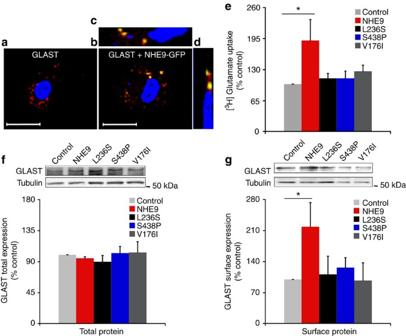Figure 9: Functional differences between NHE9 and variants revealed by glutamate uptake. (a) Subcellular localization of GLAST and NHE9 in primary cultured mouse cortical astrocytes determined by immunofluorescence confocal microscopy ( × 63 objective). Scale bars, 50 μm. GLAST (red) is distributed to vesicular compartments in untransfected astrocytes labelled with DAPI (4',6-diamidino-2-phenylindole; blue), as seen in the Merge. (b) NHE9-GFP (green) partly localizes with GLAST (red) in transfected astrocytes, as seen in the Merge. (c,d) Orthogonal views of subcellular colocalization of NHE9 with GLAST from merged image inb. (e) Glutamate uptake is elevated over control (empty vector) in astrocytes expressing NHE9-GFP but not the autism-associated variants. (f) Immunoblot (top) showing no significant change in total GLAST levels from astrocytes, after normalization to tubulin levels (graph), whereas (g) surface levels of GLAST, determined by biotinylation are elevated in cells expressing NHE9-GFP, but not autism-associated variants. Graphs represent average band intensity from densitometric scans of immunoblots from three biological replicates. GLAST levels were normalized to tubulin and shown relative to vector-transformed control. Statistical analysis was done using Student’st-test (*P<0.05). Error bars represent the average of three independent experiments with s.d. Figure 9: Functional differences between NHE9 and variants revealed by glutamate uptake. ( a ) Subcellular localization of GLAST and NHE9 in primary cultured mouse cortical astrocytes determined by immunofluorescence confocal microscopy ( × 63 objective). Scale bars, 50 μm. GLAST (red) is distributed to vesicular compartments in untransfected astrocytes labelled with DAPI (4',6-diamidino-2-phenylindole; blue), as seen in the Merge. ( b ) NHE9-GFP (green) partly localizes with GLAST (red) in transfected astrocytes, as seen in the Merge. ( c , d ) Orthogonal views of subcellular colocalization of NHE9 with GLAST from merged image in b . ( e ) Glutamate uptake is elevated over control (empty vector) in astrocytes expressing NHE9-GFP but not the autism-associated variants. ( f ) Immunoblot (top) showing no significant change in total GLAST levels from astrocytes, after normalization to tubulin levels (graph), whereas ( g ) surface levels of GLAST, determined by biotinylation are elevated in cells expressing NHE9-GFP, but not autism-associated variants. Graphs represent average band intensity from densitometric scans of immunoblots from three biological replicates. GLAST levels were normalized to tubulin and shown relative to vector-transformed control. Statistical analysis was done using Student’s t -test (* P <0.05). Error bars represent the average of three independent experiments with s.d. 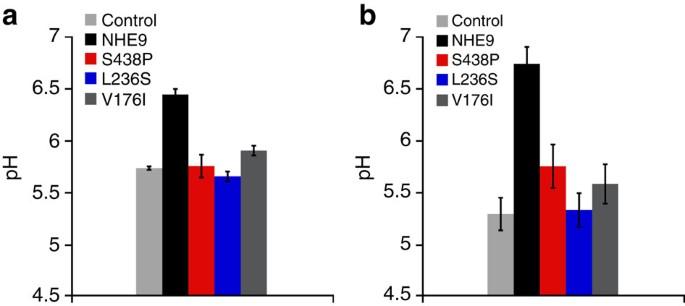Figure 10: Autism-associated NHE9 variants fail to alkalinize endosomal pH. Cells were loaded with fluorescein isothiocyanate (FITC)- and Alexa Fluor-tagged transferrin (Tf) for 55 min and internalized Tf was quantified using flow cytometry from at least 5,000 cells, in triplicate. pH was calibrated using the ratio of internalized Tf-FITC (pH sensitive) and Tf-Alexa Fluor (pH insensitive). Cells were exposed to nigericin (100 μM) and pH defined medium (pH 5.0 to pH 8.0) for calibration of pH-dependent fluorescence. (a) Expression of NHE9, but not autism-associated variants, in HEK293 cells results in alkalinization of endosomal pH. (b) NHE9 and autism-associated variants were expressed in primary mouse astrocytes, with similar results as ina. Error bars represent s.d. Full size image Figure 10: Autism-associated NHE9 variants fail to alkalinize endosomal pH. Cells were loaded with fluorescein isothiocyanate (FITC)- and Alexa Fluor-tagged transferrin (Tf) for 55 min and internalized Tf was quantified using flow cytometry from at least 5,000 cells, in triplicate. pH was calibrated using the ratio of internalized Tf-FITC (pH sensitive) and Tf-Alexa Fluor (pH insensitive). Cells were exposed to nigericin (100 μM) and pH defined medium (pH 5.0 to pH 8.0) for calibration of pH-dependent fluorescence. ( a ) Expression of NHE9, but not autism-associated variants, in HEK293 cells results in alkalinization of endosomal pH. ( b ) NHE9 and autism-associated variants were expressed in primary mouse astrocytes, with similar results as in a . Error bars represent s.d. Full size image There were two goals of this study: to assess the function of genetic variations in NHE9/ SLC9A9 associated with autism and to evaluate NHE9 as a candidate gene for ASDs in a neurobiological model. To this end, we exploited studies done with cation/proton antiporter orthologues from bacteria and yeast model organisms. Phylogenetic clustering of human NHE9 with yeast Nhx1 supports a common structural fold that relates back to the more distant bacterial orthologue, NhaA. Pairwise alignment allowed some autism-associated variants found in human NHE9 to be directly modelled on the yeast protein. In support of this, we found that conserved differences between NHE9 and Nhx1 could be swapped out without loss of function. Therefore, yeast Nhx1 serves as a convenient NHE9 surrogate for analysing a subset of variants with a conservation score of >5 ( Fig. 1a ), which may be mapped by homology with relatively high confidence. Given the rapidly increasing availability of genomic information and the prevalence of a large number of rare variants differing between individual genotypes, it will be important to have in place facile, inexpensive and rapid screening mechanisms for the functional evaluation of mutations and their potential contribution to autism and other disorders. As more autism-associated variants in NHE genes will be forthcoming, our approach will serve as a template for scoring their potential severity. A similar approach was recently used for p53 mutations, in which structure-driven assessment was used to correctly predict patient outcome [47] . Although such a detailed level of insight is not yet possible in the case of autism, our study represents an important first step towards that goal. NHE9 variants S438P and L236S, identified in autism patients with and without comorbid epilepsy, respectively, consistently scored as loss-of-function mutations in both yeast and astrocyte models. This validates predictions from the structural model placing them within highly conserved transmembrane regions of a helical bundle, central to the ion transport mechanism of the bacterial orthologues NhaA and NhaP [35] , [48] , [49] , [50] . In contrast, the Val176Ile variant, found in a patient without seizures, lies in a more variable region peripheral to the transport domain. Although it was phenotypically silent in the simpler yeast cell, functional deficits were uncovered in astrocytes, suggesting additional roles in the mammalian protein, possibly via protein interactions. For example, CHP and RACK1, two non-selective binding partners of other NHE isoforms, were also shown to bind NHE9 in a heterologous system, although the functional relevance of the interaction was not established [30] . The bacterial and eukaryotic homologues vary significantly in their amino-terminal sequences up to and including the third transmembrane helix, and the mammalian protein structure may differ from the NhaA template in this region. In this respect, it is noteworthy that cryo-electron microscopy studies of NhaP1 revealed that this archaeal sodium-proton antiporter features 13, rather than 12, transmembrane helices and a different mode of dimerization in comparison with NhaA [51] . Although more disease-associated variants would need to be analysed to determine whether such differences are unusual, we can conclude that autism-associated NHE9 mutations do impact antiporter function in vitro , and therefore may be causal to disease phenotypes. NHE9 is an eminently druggable target, and it is worth noting that considerable progress has been made in correcting loss-of-function mutations in cystic fibrosis transmembrane conductance regulator (CFTR), affecting transporter activity and trafficking using small molecule potentiators and correctors, respectively, in the treatment of cystic fibrosis [52] . Our studies provide first insights towards establishing a neurobiological role of NHE9 in a wide range of disorders, including ASD and ADHD. Whole-brain analysis of developing murine brain reveals highly specific and regulated expression of NHE9, consistent with a role in modulation of developing synapses in both neurons and astrocytes. Further, a previous study in rat models of ADHD suggested that SLC9A9 expression is proportional to the number of synapses based on a significant correlation in the expression of NHE9 and the synaptophysin [30] . Although overlapping distribution of the closely related NHE6 orthologue could result in functional redundancy, we did observe acidification of transferrin receptor (TfnR)-positive endosomes upon NHE9 knockdown in human glioma cells and, conversely, alkalinization resulting from enhanced expression in mouse astrocytes. Thus, NHE9 functions as a H + leak pathway in endosomes, acting as a brake against excessive luminal acidification. The luminal pH of sorting endosomes is critical in determining the direction of the cargo and has a crucial role in receptor desensitization, degradation and cell surface delivery of receptors upon ligand dissociation [53] . Early and recycling endosomes have more alkaline pH than late endosomes and lysosomes [54] . Alkalinization of the recycling pathway by elevated expression of NHE9 had the effect of increasing surface expression of the glutamate transporter GLAST and a consequent increase in glutamate uptake. Furthermore, this appears to be a general mechanism not specific for the astrocyte-specific transporter, given the similar observations with transferrin receptor and uptake. By extension, impairment of NHE9 function in vivo may lead to hyperacidification of endosomal lumen, as observed in the yeast model and in cultured human glioma cells. This could result in lower levels of receptors and transporters at the synaptic membranes, and decrease of synaptic clearance of glutamate, consistent with the aetiology of epilepsy and autism. Structural modelling NHE1-9, Nhx1 and NhaA belong to the CPA superfamily [15] and are classified in the monovalent CPA1 family (2.A.36) on TCDB6 database [55] . The only crystal structure available for this superfamily is the bacterial orthologue NhaA [35] . NHE9, Nhx1 and NHE1 share a sequence identity of only 14%, 15% and 10%, respectively, with NhaA. These low-sequence identities limit the alignment of sequences using standard methods. To confirm that we were using the template with the correct fold, we used the tools available on the ‘TCDB (Transporter classification database; http://www.tcdb.org/ )’ and ‘PDB (Protein Data Bank; http://www.rcsb.org/pdb/home/home.do )’. Searching the PDB starting with the NHE9 query, the first hit is the NhaA structure (1zcd). The second hit is the bile acid transporter ASBT (3zux), which shares a similar fold but has only ten transmembranes. The next hits are the transmembrane XI of the NHE1 isoform [56] . The other hits include NHE1 transmembrane XI, a putative YscO homologue (3k29; in the C-terminal region), Stathmin 4 (1sao; in the C-terminal region) and Aquaporin-4 (1ivz; 340 residues). The last hit (number 10) is Histone deacetylase 4 (2h8n; in the C-terminal region). We previously used multiple state-of-the-art approaches to construct alignments between NHE1 and NhaA [36] . An alignment of NHE9 and Nhx1 with NHE1 was constructed using the strategy described below, based on a higher shared sequence identity of 32 and 30%, respectively. The ConSeq web server ( http://conseq.bioinfo.tau.ac.il/ ) was used to generate an initial alignment. Additional pairwise alignment was calculated using the FFASO3 server [57] . Evolutionary conservation scores were calculated using the Bayesian method [58] , an empirical approach that uses Markov chain Monte Carlo methodology. Similar to the methodology used for developing the NHE1 fold, we used profile-to-profile alignments implemented in the FFASO3 server and Modeller [59] to predict protein fold [57] . Transmembrane boundaries of NHE1 guided the assignment of boundaries of the 12 transmembrane segments. Using an iterative process that included manually adjusting the alignments to reduce gaps in the transmembrane helices followed by Pfam, FFAS03 and HMAP alignments [36] , membrane topology of Nhx1 and NHE9 were predicted. Although there were some gaps in the alignments of NHE1, Nhx1 and NHE9, none of these gaps are located in the predicted transmembrane helices ( Fig. 1a ). The regions corresponding to the gaps in the alignment have no known functional roles. Evolutionarily conserved residues in both NHE9 and Nhx1 are located at the interfaces between the transmembrane segments, whereas the variable residues face the membrane lipids or are located in the extramembrane loops. The three-dimensional models are compatible with the evolutionary conservation analyses of NHE. The Consurf web server ( http://consurf.tau.ac.il/ ) was used to impose evolutionary conservation scores onto the three-dimensional models. Thus, the structural modelling procedure should provide a good approximation of helix packing in the protein core, but the conformations of some of the extramembrane loops might deviate significantly from the native structure. Plasmids A full-length mouse NHE9 cDNA was cloned into pcDNA3-EGFP using the following primers 5′-GATCATAAGCTTATGGCTGGGCAGCTTCGGTTTACG-3′ and 5′-ATGCTAGAATTCGTC CATCTGGGGTTGACCCCGAG-3′. Hin dIII and Eco RI sites were added to facilitate cloning. mNHE9-EGFP was cloned into FuGW–lentiviral vector into the Bam HI site. Stratagene’s QuikChange-Site-Directed Mutagenesis Kit was used to make the point mutations. Cell culture Cortical astrocyte cultures were prepared from P2 mouse pups [60] of mixed sex. All animal protocols were conducted according to national guidelines approved by the Johns Hopkins Animal Care and Use Committee. After dissection and removal of the meninges and blood vessels, cortices were incubated with trypsin-EDTA (0.05%, 0.2 mm) for 20 min at 37 °C. Tissue was triturated and suspended in DMEM (Invitrogen) supplemented with 10% fetal bovine serum (Invitrogen), 10% Hams F-12 and 0.24% penicillin/streptomycin (10,000 U ml −1 penicillin, 10,000 mg ml −1 streptomycin). Cells (14 ml) were plated at a density of 2.5 × 10 5 cells per ml (3 × 10 4 cells per cm 2 ) in 75 cm 2 flasks and maintained in a 5% CO 2 incubator at 37 °C. The growth medium was completely exchanged with fresh medium twice a week until cells were 90% confluent (9–10 days). Quantitative real-time PCR mRNA was isolated using RNeasy Mini kit from Qiagen following the manufacturer’s instructions. RNA was treated with DNase I (1 unit for 1 μg RNA; Roche) following which the DNase was inactivated by EDTA (final concentration of 3 mM) at 65 °C for 10 min. High-capacity RNA-cDNA kit (Applied Biosystems, Carlsbad, CA; catalogue number 4387406) was used to make cDNA from RNA, following the manufacturer’s instructions. Gene expression levels were measured by quantitative real-time PCR using Taqman gene expression assays (The Step One Plus Real-Time PCR System, Applied Biosystems). The gene expression assays used were Mm00626012_m1 ( SLC9A9 solute carrier family 9 (sodium/hydrogen exchanger), member 9) and Mm00555445_m1 ( SLC9A6 solute carrier family 9 (sodium/hydrogen exchanger), member 6). Mm03928990_g1 (Rn18s, 18S ribosomal RNA) and Mm99999915_g1 (GAPDH, glyceraldehyde-3-phosphate dehydrogenase) were our endogenous control. Each experiment had three technical replicates and was repeated three times independently (biological replicates) to account for intra- and interassay variances, respectively. Ct values were used for all manipulations and were first normalized to endogenous control levels by calculating the ΔCt for each sample. Values were then calculated relative to control to generate a ΔΔCt value. Fold change was calculated using the formula Fold Change (RQ)=2 −ΔΔCt . Statistical significance was determined based on the biological replicates and the s.d. (Student’s t -test) plotted, representing the variance between the biological replicates. Functional complementation in yeast All Saccharomyces cerevisiae strains used were derivatives of BY4742 (ResGen; Invitrogen). The complementation studies [33] and measurement of vacuolar pH [33] , [38] , [61] were done as follows. Yeast strains, media and growth conditions: Derivatives of BY4742 S. cerevisiae strains were grown in synthetic complete medium to saturation, washed three times in water and used to seed 200 μl of APG medium (arginine phosphate glucose, a synthetic minimal medium containing 10 mM arginine, 8 mM phosphoric acid, 2% (w/v) glucose, 2 mM MgSO 4 , 1 mM KCl and 0.2 mM CaCl 2 , and trace minerals and vitamins) to a starting attenuance of 0.05 OD 600 units per ml. Phosphoric acid was used to adjust the pH to 4.0 or 2.7. NaCl, KCl or hygromycin was added as indicated and growth was monitored by measuring OD 600 after culturing for 24 h at 30 °C. Measurement of vacuolar pH: Cells were grown for 18 h at 30 °C in APG growth medium, absorbance readings were taken at 600 nm to measure growth, and cultures were then incubated with 50 μM BCECF (2′,7′-bis-(2-carboxyethyl)-5(6)-carboxyfluorescein)-acetoxymethyl ester) at 30 °C for 20 min, washed and suspended in APG medium. Normalized background-subtracted fluorescence emission values at 485 nm were calculated (NI 485 (normalized intensity at 485 nm)) using fluorescence intensity and absorbance readings taken at 485 and 600 nm, respectively. A calibration curve of the ratio of fluorescence intensity values versus pH was obtained for each yeast strain at the end of every experiment and vacuolar pH values were determined by incubating yeast cultures in 200 μl of experimental medium, titrated to five different pH values within the range of 4.0–8.0 using 1 M NaOH (refs 33 , 38 , 61 ). CPY secretion: Yeast cultures were seeded in synthetic complete media to a starting OD 600 of 0.05 ml −1 and grown at 30 °C for 20 h. Cells (1.5 OD 600 ) were centrifuged for 2 min and 600 μl of the supernatants were applied to Immobilon (Millipore) membranes using a slot-blot apparatus (Schleicher & Schuell Manifold II). After drying the membrane overnight, CPY was detected by immunoblotting using monoclonal anti-CPY antibody (Molecular Probes; 1:1,000 dilution). Immunofluorescence Cultured glial cells on coverslips were pre-extracted with PHEM buffer (60 mM PIPES, 25 mM HEPES, 10 mM EGTA, and 2 mM MgCl 2 , pH 6.8) containing 0.025% saponin for 2 min, then washed twice for 2 min with PHEM buffer containing 0.025% saponin and 8% sucrose. The cells were fixed with a solution of 4% paraformaldehyde and 8% sucrose in PBS for 30 min at room temperature and blocked with a solution of 1% BSA and 0.025% saponin in PBS for 1 h. Primary antibodies were diluted in 1% BSA and incubated with the cells for 1 h. Alexa Fluor 568 goat anti-rabbit IgG (Invitrogen) and Alexa Fluor 568 (Invitrogen) goat anti-mouse IgG were used at a 1:1,000 dilution for 30 min. Cells were mounted onto slides using Dako Fluorescent Mounting Medium. Slides were imaged on a Zeiss LSM510-Meta confocal microscope. Fractional colocalization was determined from Mander’s coefficient, which measures the direct overlap of green and red pixels in the confocal section. The value range is from 0 to 1 (0, no colocalization; 1, all pixels colocalize). The Mander’s coefficient is independent of differences in signal intensity between the two channels. Steady-state transferrin uptake and pH measurement Astrocytes or HEK293 cells were rinsed and incubated in serum-free medium for 30 min to remove any residual transferrin and then were exposed to 100 μg ml −1 transferrin conjugated with Alexa Fluor 568 or 633 (Invitrogen) at 37 °C for 55 min. Uptake was stopped by chilling the cells on ice. External transferrin was removed by washing with ice-cold serum-free DMEM and PBS, whereas bound transferrin was removed by an acid wash in PBS at pH 5.0 followed by a wash with PBS at pH 7.0. Surface-bound transferrin (less than 5% of total) was determined with a parallel sample incubated on ice and was used for background subtraction. The fluorescence intensity of internalized transferrin was measured for at least 5,000 cells by flow cytometry using the FACSAria (BD Biosciences, San Jose, CA) instrument and the average intensity of the cell population was recorded. Glutamate uptake assay Glutamate uptake into primary astrocytes was measured using 0.5 μM l -glutamate and 0.3 μCi l -[ 3 H]glutamate per sample (cold:radioactive=99:1) [62] . Cells were first washed and pre-incubated at 25 °C for 10–20 min in Na + buffer (5 mM Tris–HCl, pH 7.2, 10 mM HEPES, 140 mM NaCl, 2.5 mM KCl, 1.2 mM CaCl 2 , 1.2 mM MgCl 2 , 1.2 mM K 2 HPO 4 and 10 mM D -glucose). Glutamate uptake reaction was initiated by incubating cells for 5 min at 37 °C in Na + uptake buffer (0.5 μM l -glutamate and 0.3 μCi l -[3H]glutamate per sample in Na + buffer), followed by two quick washes with ice-cold Na + -free assay buffer (5 mM Tris–HCl, pH 7.2, 10 mM HEPES, 140 mM Choline-Cl, 2.5 mM KCl, 1.2 mM CaCl 2 , 1.2 mM MgCl 2 , 1.2 mM K 2 HPO 4 and 10 mM D -glucose). NaOH (0.1 N) solution was then used to lyse the cells and radioactivity was measured using a scintillation counter. Background radiation was subtracted for each sample separately by incubating the cells for 0 min (immediate removal following addition of hot uptake buffer) on ice followed by quick washes with ice-cold Na + -free assay buffer. Western blotting and cell surface biotinylation Surface proteins labelled with biotin [10] . Briefly, cells were washed three times with ice-cold PBS and incubated with 1 mg ml −1 Sulpho-NHS-LC-biotin in PBS at 4 °C for 20 min. Excess NHS groups were quenched using 100 mM glycine followed by three washes with PBS. Nonidet P-40 (1% ), with protease inhibitor cocktail (Roche), was used to lyse cells and then centrifuged for 10 min at 14,000 r.p.m. at 4 °C. Protein supernatants were mixed with 120 μl of immobilized Neutravidin beads and incubated at 4 °C overnight with gentle rotation. Beads collected by centrifugation were washed three times with lysis buffer, and surface proteins labelled with biotin were separated by SDS–PAGE and analysed by immunoblotting. Blots were cropped to show relevant bands; all full-sized blots are shown in Supplementary Fig. S1 . How to cite this article: Kondapalli, K. C. et al. Functional evaluation of autism-associated mutations in NHE9. Nat. Commun. 4:2510 doi: 10.1038/ncomms3510 (2013).